Orbital-selective metal–insulator transition and gap formation aboveTCin superconducting Rb1−xFe2−ySe2 Understanding the origin of high-temperature superconductivity in copper- and iron-based materials is one of the outstanding tasks of current research in condensed matter physics. Even the normal metallic state of these materials exhibits unusual properties. Here we report on a hierarchy of temperatures T c < T gap < T met in superconducting Rb 1− x Fe 2− y Se 2 observed by THz spectroscopy (T c =critical temperature of the superconducting phase; T gap =temperature below which an excitation gap opens; T met =temperature below which a metallic optical response occurs). Above T met =90 K the material reveals semiconducting characteristics. Below T met a coherent metallic THz response emerges. This metal-to-insulator-type, orbital-selective transition is indicated by an isosbestic point in the temperature dependence of the optical conductivity and dielectric constant at THz frequencies. At T gap =61 K, a gap opens in the THz regime and then the superconducting transition occurs at T c =32 K. This sequence of temperatures seems to reflect a corresponding hierarchy of the electronic correlations in different bands. The normal state above the superconducting transition temperatures in copper- and iron-based high-temperature superconductors is thought to provide important information on the superconducting state itself, and very often exhibits unusual properties. These properties have been interpreted as ordering phenomena of spin or charge carriers before the formation of the superconducting state [1] , [2] , [3] , [4] , [5] . Recently, an orbital-selective Mott transition has been suggested to occur in the normal-state phase of iron-selenide superconductors [6] , [7] , [8] , [9] , where some of the five d orbitals independently undergo metal-to-insulator-like transitions. The selenide iron-based superconductors offer the opportunity to explore superconductivity all the way from binary FeSe with T c =8 K (ref. 10 ) and the alkaline-doped A 1− x Fe 2− y Se 2 ( A =K, Rb and Cs) with T c =32 K (refs 11 , 12 , 13 ) to epitaxial single-layer FeSe films with T c =65 K (refs 14 , 15 ). Critical temperatures up to 46 K are obtained by intercalation [16] , [17] , [18] and 48 K by applying pressure [19] , [20] . Superconductivity in A 1− x Fe 2− y Se 2 was shown to occur only in single crystals, where a mesoscopic separation into a superconducting phase with T c ≈32 K and an antiferromagnetic phase with a Néel temperature T N ≈550 K has been established [11] , [12] , [13] , [21] , [22] , [23] , [24] (see Fig. 1c ). The superconducting phase is electron-doped with about 0.15 electrons per Fe atom [23] . Angle-resolved photoemission spectroscopy (ARPES) studies determined the Fermi-surface topology with large electron-like Fermi sheets δ at the M points and small electron pocket κ at the Γ point [25] (see Fig. 1d ). Isotropic superconducting gaps of 2Δ ≃ 16 and 20 meV were reported around the κ and δ pockets, respectively [25] . In addition, a small gap 2Δ ≃ 2 meV was observed by scanning tunnelling spectroscopy [21] . Recently, the normal state of the superconducting phase was reported to exhibit an orbital-selective metal-to-insulator transition [7] observed by ARPES at about 100 K (ref. 6 ). Moreover, interphase correlations between superconducting and antiferromagnetic layers were predicted to reduce T c from a hypothetical 65 K to the actually observed value of 32 K owing to proximity effects [26] (see Fig. 1e ). 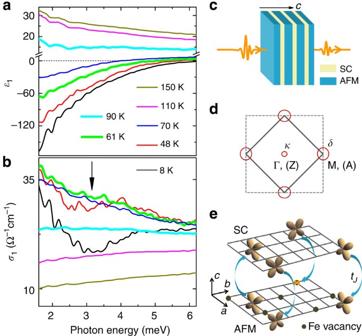Figure 1: Photon energy dependence of dielectric constant and optical conductivity. (a,b) Dielectric constantε1and optical conductivityσ1of Rb0.74Fe1.60Se2in the THz spectral region at various temperatures. The arrow inbindicates the formation of a gap at about 3 meV belowTgap≈61 K. (c) Schematic sketch of the THz transmission experiment on the sample consisting of superconducting (SC) and antiferromagnetic (AFM) layers24. (d) Sketch of Brillouin zone and Fermi surface25. (e) Illustration of interphasedxz/dyzelectron hopping (tJ) between Fe atoms from SC and from AFM layers (adapted from Huanget al.26). Figure 1: Photon energy dependence of dielectric constant and optical conductivity. ( a , b ) Dielectric constant ε 1 and optical conductivity σ 1 of Rb 0.74 Fe 1.60 Se 2 in the THz spectral region at various temperatures. The arrow in b indicates the formation of a gap at about 3 meV below T gap ≈61 K. ( c ) Schematic sketch of the THz transmission experiment on the sample consisting of superconducting (SC) and antiferromagnetic (AFM) layers [24] . ( d ) Sketch of Brillouin zone and Fermi surface [25] . ( e ) Illustration of interphase d xz / d yz electron hopping ( t J ) between Fe atoms from SC and from AFM layers (adapted from Huang et al. [26] ). Full size image In this article we report on terahertz (THz) spectroscopy studies on superconducting Rb 1− x Fe 2− y Se 2 . The temperature dependence of the optical conductivity and dielectric constant exhibits an isosbestic point at T met =90 K indicating a metal-to-insulator-type, orbital-selective transition. At T gap =61 K, a gap-like suppression of the optical conductivity is observed and is followed by the occurrence of the superconducting transition at T c =32 K. This hierarchy of temperatures T c < T gap < T met seems to imply that the quasiparticles in the d xy band are more strongly correlated. Dielectric constant and optical conductivity Figure 1a,b shows the dielectric constant ε 1 and the optical conductivity σ 1 as a function of incident photon energy, respectively, derived from the time domain THz transmission signal (see Methods) for selected temperatures across the three characteristic temperatures T c =32 K, T gap =61 K and T met =90 K. From room temperature down to T met =90 K, ε 1 is positive and slightly increases towards lower temperatures, which is characteristic of a semiconducting optical response ( Fig. 1a ). Below 90 K, the dielectric constant becomes negative with a zero-crossing point from 2.5 meV at 80 K to 6.5 meV at 8 K. This is a fingerprint of a metallic system, and the observed zero-crossing points in ε 1 correspond to the reported screened plasma frequencies [22] , [27] , [28] , [29] . Similar observations, namely, the smooth transition from an insulating to a metallic state, are made in the frequency dependence of the optical conductivity σ 1 for several temperatures ( Fig. 1b ). Above T met =90 K, σ 1 is low and almost energy independent, indicating a semiconducting behaviour of quasi-localized charge carriers, while below this characteristic temperature a metallic response evolves with an increase of σ 1 towards lower energies. In contrast to the monotonous decrease of ε 1 with decreasing temperature, σ 1 decreases for temperatures below T gap =61 K and below energies of 5 meV. Towards lower temperatures, a gap-like feature (see arrow in Fig. 1b ) evolves with a minimum in σ 1 close to E gap ~3 meV. Its temperature dependence is shown as an inset to Fig. 2b . 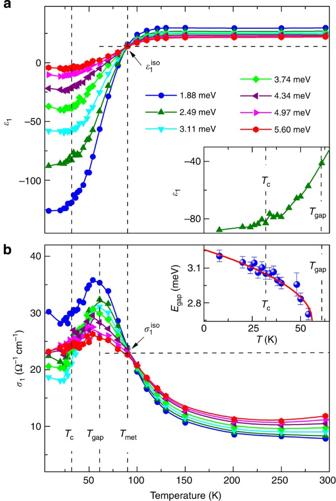Figure 2: Temperature dependence of dielectric constant and optical conductivity. (a,b) Dielectric constantε1and optical conductivityσ1as a function of temperature at different photon energies. The characteristic temperatures and the isosbestic points are indicated by dashed lines. Inset toa, temperature dependence ofε1at 2.49 meV aroundTc. Inset tob, temperature dependence of the gap energyEgap(the solid line is drawn to guide the eyes). Error bars indicate uncertainties larger than the data point size. The gap energy appears to increase continuously across T c =32 K. Furthermore, the spectra of ε 1 and σ 1 do not exhibit drastic changes at T c =32 K, well below T gap =61 K. Figure 2: Temperature dependence of dielectric constant and optical conductivity. ( a , b ) Dielectric constant ε 1 and optical conductivity σ 1 as a function of temperature at different photon energies. The characteristic temperatures and the isosbestic points are indicated by dashed lines. Inset to a , temperature dependence of ε 1 at 2.49 meV around T c . Inset to b , temperature dependence of the gap energy E gap (the solid line is drawn to guide the eyes). Error bars indicate uncertainties larger than the data point size. Full size image Isosbestic points To analyse these striking temperature-induced changes of the optical response in more detail, Fig. 2a,b shows the dielectric constant and the conductivity as a function of temperature for several photon energies. At high temperatures, the dielectric constant is positive and almost temperature independent. At the same time the optical conductivity is low and increases gradually with decreasing temperature. This increase of σ 1 becomes stronger when T met =90 K is approached from above, while the dielectric constant ε 1 decreases and becomes negative below T met , signalling metallic behaviour. This metal-to-insulator-like transition is indicated by two sharp isosbestic points where all curves intersect and are therefore strictly frequency independent. At these points, the dielectric constant and optical conductivity take the values =14 and =22 Ω −1 cm −1 , respectively. The increase of the optical conductivity for decreasing temperature terminates at T gap =61 K, and after which σ 1 starts to decrease, thus leading to a pronounced maximum. This signals the opening of a gap (see Fig. 1b ) far above the superconducting transition temperature, T c =32 K. Indeed, the superconducting transition at T c =32 K leads to a weak kink (see inset of Fig. 2a for ε 1 ) and a subsequent levelling off of both quantities. The existence of isosbestic points in the plots of ε 1 ( T , ω ) versus T and σ 1 ( T , ω ) versus T , respectively, allows one to determine their frequency dependences as ε 1 ( T , ω )= ε 1 ( T , ω 0 )+(1/ ω −1/ ω 0 ) E 1 ( T ) and σ 1 ( T , ω )= σ 1 ( T , ω 0 )+( ω − ω 0 ) S 1 ( T ) in the vicinity of these points [30] , [31] (see Methods). Using the parameters E 1 ( T ) and S 1 ( T ) ( Fig. 3c,d ), which were obtained by fitting the spectra as shown in Fig. 3a,b , the validity of the approximations is demonstrated in Fig. 3e,f . All curves are shown to collapse onto the one for ω 0 =1.88 meV. We note that the observed frequency dependencies can be applied to both temperature regimes, above and below T met =90 K. Given the intrinsic phase separation of the compound, these frequency dependences are excellent low-frequency parametrizations of the actual optical response functions. Such well-defined frequency dependencies have not been observed in previous studies [27] , [28] , [29] and are valid only in the vicinity of sharp isosbestic points [30] . 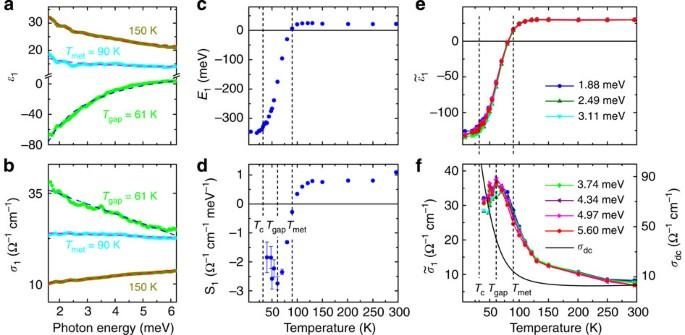Figure 3: Scaling of the dielectric constant and the optical conductivity. (a,b) Fits of the dielectric constant usingε1(ω)~E1/ωandσ1(ω)~S1ωfor selected temperatures, respectively. (c,d) Temperature dependences of the respective fit parametersE1andS1. Error bars indicate uncertainties larger than the data point size. (e,f) Scaled dielectric constant=ε1−(1/ωi−1/ω0)E1and optical conductivity=σ1−(ωi−ω0)S1for different frequenciesωi. The curves collapse on the ones forω0=1.88 meV (see Methods). For comparison, the temperature dependence of thedcconductivityσdcis shown inf(scale on the right). Figure 3: Scaling of the dielectric constant and the optical conductivity. ( a , b ) Fits of the dielectric constant using ε 1 ( ω )~ E 1 / ω and σ 1 ( ω )~ S 1 ω for selected temperatures, respectively. ( c , d ) Temperature dependences of the respective fit parameters E 1 and S 1 . Error bars indicate uncertainties larger than the data point size. ( e , f ) Scaled dielectric constant = ε 1 −(1/ ω i −1/ ω 0 ) E 1 and optical conductivity = σ 1 −( ω i − ω 0 ) S 1 for different frequencies ω i . The curves collapse on the ones for ω 0 =1.88 meV (see Methods). For comparison, the temperature dependence of the dc conductivity σ dc is shown in f (scale on the right). Full size image The change from insulating to metallic behaviour is reflected by the sign change of E 1 ( T ) and S 1 ( T ) from positive to negative at T met =90 K. While E 1 ( T ) saturates below T c , S 1 ( T ) drops strongly with decreasing temperature until a minimum is reached at T gap =61 K. The gap-like suppression of the optical conductivity below T gap leads to a clear deviation from a linear frequency dependence (see larger error bars in Fig. 3d ), implying that the frequency dependence of σ 1 derived above does not hold below a temperature of about 40 K. The emergence of a metallic optical response below T met =90 K can be understood as a consequence of an orbital-selective Mott transition, which was proposed to explain the result of a recent ARPES study in A x Fe 2− y Se 2 with A =K, Rb (ref. 6 ). Specifically, for a doping of 0.15 electrons per Fe, the investigation of a five-orbital Hubbard model discovered an orbital-selective Mott transition where the d xy band contributes to the metallic properties only below a temperature of about 100 K, while the d xz / d yz bands retain their metallic features both below and above 100 K (refs 6 , 7 ). This scenario closely follows the general physical picture of strong orbital differentiation with a low coherence temperature [32] . The collapsed optical conductivity curve in Fig. 3f exhibits the same temperature dependence as the ARPES spectral weight associated with the d xy band of the electron pocket at the M point [6] . Thus, we conclude that the optical conductivity probes predominantly the d xy band and signals a Mott transition of this band at the temperature of the isosbestic point T met =90 K. The pronounced orbital differentiation [8] , [9] of Rb 1− x Fe 2− y Se 2 manifests itself through highly orbital-dependent mass renormalizations of about 10 for the d xy band and about 3 for the d xz / d yz bands [6] . Owing to the significantly stronger correlation strength, the lifetime of quasiparticles in the d xy band is much more susceptible to temperature than in the other bands. This leads to a selective reduction of the d xy quasiparticle peak, which effectively eliminates its contribution to transport processes with increasing temperature. The lighter d xz / d yz quasiparticles will, however, dominate the transport properties. Indeed, no anomaly is visible in the dc resistivity σ dc at T met ≈90 K in Fig. 3f (ref. 13 ). The optical conductivity is expected to be governed by all quasiparticles, but instead it determines the temperature dependence of the strongly renormalized d xy charge carriers. To explain the orbital differentiation of the optical conductivity, we have to consider the special morphology of the phase-separated system. Huang et al. [26] investigated effects of interlayer hopping at the interface of the superconducting and the antiferromagnetic phases in the d xz / d yz channels (sketched in Fig. 1e ) and found that the resulting distortions of the Fermi surfaces effectively reduce T c . We assume that these incoherent hopping processes via the d xz / d yz bands lead to large scattering rates in the optical response of the corresponding quasiparticles of the d xz / d yz bands. By contrast, the d xy channel remains almost unaffected by the proximity effect and reveals its metallic optical response at low frequencies via its larger mass normalization. Without the distortions of the Fermi surface induced by the vicinity of the antiferromagnetic phase a value of T c as high as 65 K is estimated [26] . This scenario is supported by the formation of a gap already below T gap =61 K in the d xy -dominated optical conductivity. The upper bound for the gap at 3.2 meV must be compared with the gap value of 2Δ ≃ 2 meV found in a scanning tunnelling microscopy study on films of K 1− x Fe 2− y Se 2 (ref. 21 ). The fact that the conductivity is not completely suppressed below 3.2 meV points towards an anisotropic nature of this low-frequency gap. Our observations provide strong support for the existence of an orbital-selective Mott transition, and also point to the possibility of orbital-selective superconducting properties [33] . The appearance of a gap in the d xy -dominated optical conductivity at T gap =61 K in superconducting Rb 1− x Fe 2− y Se 2 may be compared with the reported opening of a gap below 65 K in single-layer FeSe films, which was interpreted as an indication for the onset of superconducting fluctuations at this temperature [14] . Given the similarity of the electronic band structures of FeSe monolayer films and Rb 1− x Fe 2− y Se 2 (ref. 14 ), we predict that the highest possible value of T c in Fe selenide systems is determined by the correlated quasiparticles in the d xy channel. Crystal growth Pure Rb and polycrystalline FeSe (99.75%), preliminarily synthesized from the high-purity elements (99.985% Fe and 99.999% Se) were used as starting materials. Crystals of Rb 0.74 Fe 1.60 Se 2 were grown using the Bridgman method from the starting composition corresponding to the Rb 0.8 Fe 2 Se 2 stoichiometry. The samples have been soaked at 1,070 °C for 5 h. The cooling rate is 3 mm h −1 (ref. 13 ). Crystals of the same sample batch were investigated by magnetization [13] , resistivity, nuclear magnetic resonance [23] , muon spin rotation and scanning near-field microscopy [24] . Scaling analysis around the isosbestic points In general, an isosbestic point is an intersection point of a family of n curves f ( x , p i ) , i=1 , 2 , …, n in the plot of f ( x ) (refs 30 , 31 ). Since isosbestic behaviour is observed only in a certain parameter range around a particular value p 0 , we can expand around p 0 as f ( x , p i ) =f ( x , p 0 )+( p i − p 0 ) F 1 ( x , p 0 ) +O [( p i − p 0 ) 2 ], where F 1 ( x )=∂ f /∂ p| p=p0 is a function of x only. The scaling of f ( x , p i ) is calculated as ( x , p i )= f ( x , p i )−( p i − p 0 ) F 1 ( x , p 0 )= f ( x , p 0 ) +O [( p i − p 0 ) 2 ]. The validity of the expansion approximation is verified by ( x , p i ) curves for different p i collapsing on a single curve. Here x ≡ T ; f ≡ ε 1 and σ 1 ; and ; F 1 ≡ E 1 and S 1 ; p i ≡ 1/ω i and ω i . THz spectroscopy measurements Time domain THz transmission measurements were carried out on a single crystal with the THz electric field parallel to the ab plane in the spectral range 1–10 meV using a TPS spectra 3000 spectrometer (TeraView Ltd.). Transmission and phase shift were obtained from the Fourier transformation of the time domain signal. The dielectric constant and optical conductivity were calculated from the transmission and phase shift by modelling the sample as a single-phase dielectric slab. The single crystal for optical measurements was prepared with a thickness of about 45 μm and a cross-section of about 5 mm 2 . A 4 He-flow magneto-optical cryostat (Oxford Instruments) was used to reach the temperature range 8–300 K. How to cite this article: Wang, Z. et al. Orbital-selective metal–insulator transition and gap formation above T C in superconducting Rb 1− x Fe 2− y Se 2 . Nat. Commun. 5:3202 doi: 10.1038/ncomms4202 (2014).